An ultra-sensitive resistive pressure sensor based on hollow-sphere microstructure induced elasticity in conducting polymer film Pressure sensing is an important function of electronic skin devices. The development of pressure sensors that can mimic and surpass the subtle pressure sensing properties of natural skin requires the rational design of materials and devices. Here we present an ultra-sensitive resistive pressure sensor based on an elastic, microstructured conducting polymer thin film. The elastic microstructured film is prepared from a polypyrrole hydrogel using a multiphase reaction that produced a hollow-sphere microstructure that endows polypyrrole with structure-derived elasticity and a low effective elastic modulus. The contact area between the microstructured thin film and the electrodes increases with the application of pressure, enabling the device to detect low pressures with ultra-high sensitivity. Our pressure sensor based on an elastic microstructured thin film enables the detection of pressures of less than 1 Pa and exhibits a short response time, good reproducibility, excellent cycling stability and temperature-stable sensing. Electronic skin [1] , [2] , [3] , [4] , [5] mimics the functions of natural skin by transducing physical variables such as pressure [6] , [7] , [8] , [9] , [10] , temperature [11] , moisture [12] and other physiological parameters into electronic signals [13] , [14] , [15] , [16] , with applications in robotics and medicine. Promising routes towards the development of pressure sensors with sensitivity on a par with human skin have been demonstrated in recent years, with capabilities in both the low-pressure regime (<10 kPa, approximating gentle touch) and the medium-pressure regime (10–100 kPa, enabling object manipulation) [7] , [8] , [17] , [18] , [19] . The need to develop pressure sensors that can mimic and surpass the subtle pressure sensing properties of natural skin requires the rational design of innovative materials and devices [7] , [19] . Piezoresistive sensors transduce mechanical strain into an impedance change and are widely used due to their simple read-out mechanism, sensitivity to both pressure and flexion [19] and potentially high pixel density [20] . Very recently, a resistive-type pressure sensor made of self-healing materials was demonstrated, showing that the self-healing capability of natural skin could be mimicked in artificial electronic skins [21] . Many of the reported resistive-type sensors function based on bulk piezoresistivity and employ composites of insulating polymers and conductive additives as the active layer [22] . However, the performance of these devices is limited by the bulk mechanical properties of the rubbers used, for instance, poor sensitivity due to a relatively large modulus, creep and slow response time due to viscoelasticity and poor signal stability as a function of temperature due to thermal expansion. Alternatively, a related sensing mechanism involves utilizing the contact resistance between the electrode and a conducting film. These types of sensors offer the potential advantages of high sensitivity, a rapid transient response, a large working range and small temperature dependence [19] , [23] . However, such kind of devices show unstable contact in the ultra-low-pressure regime or high loading speed due to the lack of elastic component, and the limit of detection for commercially available devices is typically in the range of a few grams [24] , [25] . In the present research, we describe a new type of piezoresistive sensor in which the active layer is both conductive and elastic that imparts ultra-high sensitivity and reproducible sensing characteristics. The key innovation of our material design, elastic microstructured conducting polymer (EMCP), consists of interconnected hollow-sphere structures of polypyrrole (PPy) that were prepared through a multiphase synthesis technique. It is worth to note that dense PPy is stiff and brittle due to its rigid conjugated-ring backbone. However, by forming a spherical shell geometry, inherently brittle nanostructured materials can be made to exhibit tunable effective elastic modulus that are capable of withstanding large effective strains and stresses [26] . The hollow-sphere structure employed in our study enabled the PPy to elastically deform and recover upon the application and release of external pressure (as shown in the schematic illustration in Fig. 1a ), thereby promoting the contact stability of the pressure sensor and endowing the device with stable and reproducible sensing performance. Various hollow-structured materials have been used previously in capacitance and bulk piezoresistivity pressure sensors, but they were composed of millimeter-sized voids and exhibited notably poor sensing performance in the low-pressure regime [27] , [28] . For example, resistive sensors employing a PPy-coated polyurethane foam exhibited a sensitivity of ~0.00283, kPa −1 (with a loading of 3.46 kPa) [28] , which were 20–30 times less sensitive than that attained in the present work. Capacitive sensors based on polyolefin foam were demonstrated, but are 25 times less pressure sensitive and exhibit response/relaxation times that are 20–200 times slower than those attained in this work [29] . 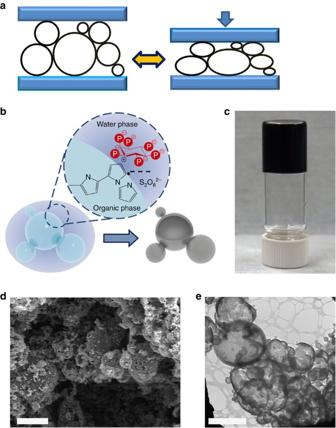Figure 1: EMCP synthesis and microstructure characterization. (a) Schematic of the structural elasticity of the hollow-sphere-structured PPy. (b) Schematic illustration of the interphase synthesis mechanism of PPy hydrogels with hollow-sphere microstructures. (c) Digital photograph of a PPy hydrogel. (d) Typical scanning electron microscope (SEM) image of the PPy thin film, scale bar: 10 μm. (e) Transmission electron microscopy (TEM) image of PPy revealing its interconnected hollow-sphere structure, scale bar: 1 μm. Figure 1: EMCP synthesis and microstructure characterization. ( a ) Schematic of the structural elasticity of the hollow-sphere-structured PPy. ( b ) Schematic illustration of the interphase synthesis mechanism of PPy hydrogels with hollow-sphere microstructures. ( c ) Digital photograph of a PPy hydrogel. ( d ) Typical scanning electron microscope (SEM) image of the PPy thin film, scale bar: 10 μm. ( e ) Transmission electron microscopy (TEM) image of PPy revealing its interconnected hollow-sphere structure, scale bar: 1 μm. Full size image Material synthesis and structural characterization The EMCP thin film was fabricated by mixing and casting a bi-component PPy gel precursor in a Petri dish. A multiphase reaction mechanism was employed to achieve the hollow-sphere morphology of the PPy, as schematically illustrated in Fig. 1b . In a typical synthesis, an aqueous solution of oxidative reagent (solution A) was mixed with a solution containing a mixture of the pyrrole monomer, isopropanol and phytic acid (solution B). The phytic acid molecule acts as both of the roles as dopant and crosslinker of PPy ( Supplementary Fig. S1 ). An emulsion formed upon mixing due to the phase separation between the organic and aqueous components, which was confirmed by dynamic light scattering measurements ( Supplementary Fig. S2 ). With the polymerization of PPy, the solution underwent a colour change from light brown (the colour of phytic acid) to black (the colour of PPy) and gelated in ~3 s (ref. 30 ). After exchanging the impurities with deionized water, the PPy gel became a hydrogel as shown in Fig. 1c . The chemical structure of the as-synthesized PPy was analysed by fourier transform infrared spectroscopy (FTIR), and the resulting spectrum was identical to that of typical PPy ( Supplementary Fig. S3 ). This facile solution gelation mechanism allowed us to fabricate large area thin films as large as 255 cm 2 by a simple casting process ( Supplementary Fig. S4 ). Scaling to even larger area should be straightforward using blade coating or other large area-coating methods [31] . A scanning electron microscope image ( Fig. 1d ) shows the three-dimensional (3D) porous foam morphology of the dried PPy film. The PPy foam consists of interconnected spheres with polydisperse diameters ranging from hundreds of nanometres to several microns. Further investigation by transmission electron microscopy revealed that the PPy possessed a hollow-sphere structure with a thin-shell thickness of ~50 nm, as shown in Fig. 1e . The conductivity of the as-synthesized PPy (pressed into pellets) was measured to be 0.5 S· cm −1 using a standard four-point probe method at room temperature. Our multiphase synthetic approach is general and tunable such that PPy thin films with hollow spheres and solid spheres of different diameters, size dispersions and shell thickness can be prepared by choosing different solvents for solution B, including 1-butanol, t -butanol, s -butanol and t -amyl alcohol ( Supplementary Fig. S5 ). Elasticity of the EMCP To assess the mechanical properties of the PPy film, we measured the compressive stress ( σ , the applied force divided by the film area) as a function of strain ( ε , the compressed distance divided by the film thickness). 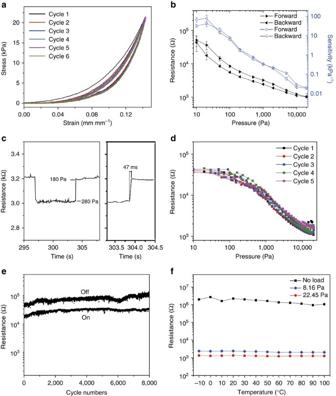Figure 2: Mechanical and pressure-sensing characterization of EMCP. (a) Six consecutive compression tests on the EMCP thin film. (b) Resistance response and pressure sensitivity of the EMCP pressure sensor. The error bars represent one standard deviation. (c) Instant response of the EMCP pressure sensor, which exhibits response times of 50 ms (the right figure shows the magnified curve of the left one). (d) First five cycles of the piezoresistance of the device. (e) Resistance of the EMCP pressure sensor over 8,000 cycles. (f) Temperature-dependent resistance response of the device. Figure 2a presents a plot of σ versus ε for six loading cycles of a typical PPy film sample with a thickness of ~181 μm and an area of 1 cm 2 . The maximum σ and ε values in the loading cycles were ~20 kPa and 14%, respectively. We define an effective elastic modulus ( E eff ) as the slope of the stress versus strain plot, which is influenced by the materials properties, morphology and roughness of the EMCP. The EMCP exhibited an E eff that was very low at low pressures and increased with compression. The E eff at 5 kPa was 0.19 MPa, which is similar to a typical low-modulus elastomer such as polydimethylsiloxane (PDMS) [32] . The E eff normalized by the density was calculated to be ~1.11 MPa cm 3 g −1 (at 5 kPa), which is lower than the many of the values reported for the modulus of foams based on polymers [33] and carbon nanotubes [34] . The first cycle of compression induced a slight plastic deformation, whereas subsequent cycles were effectively indistinguishable. Output drift during the first several cycles is common in resistive pressure sensors, and often, a ‘preconditioning’ step can be implemented, during which a large force is applied so that subsequent measurements will be reproducible [35] . Hysteresis in both mechanical and electrical properties was quantified as the maximum difference between the loading and unloading curve divided by the full-scale output. The hysteresis of EMCP was found to be ~11.0% at a maximum pressure of 20 kPa ( Supplementary Fig. S6 ), which is much lower than the hysteresis observed for conductive foams [26] , [27] . The hysteresis is reduced at lower applied strains, demonstrating the effectiveness of the sensor in the low-pressure regime [36] . Hysteresis in the mechanical properties is caused by viscoelasticity of the material, which can be characterized using dynamic mechanical analysis. Dynamic mechanical analysis measurements were conducted at 25 °C over a frequency range from 0.1 to 200 Hz ( Supplementary Fig. S7 ). The storage and loss moduli were similar to that observed in soft polymer foams [37] . The loss tangent is defined as the loss modulus divided by the storage modulus, and can be used as a measure of hysteresis [38] . The loss tangent varied from ~0.1 to 0.2 throughout the measured frequency range, which is consistent with the hysteresis value of 11.0% extracted from stress–strain data. Foams composed of CNTs [39] , graphite [40] and polymers [37] exhibit similar loss tangent values. Figure 2: Mechanical and pressure-sensing characterization of EMCP. ( a ) Six consecutive compression tests on the EMCP thin film. ( b ) Resistance response and pressure sensitivity of the EMCP pressure sensor. The error bars represent one standard deviation. ( c ) Instant response of the EMCP pressure sensor, which exhibits response times of 50 ms (the right figure shows the magnified curve of the left one). ( d ) First five cycles of the piezoresistance of the device. ( e ) Resistance of the EMCP pressure sensor over 8,000 cycles. ( f ) Temperature-dependent resistance response of the device. Full size image Piezoresistance property of EMCP The EMCP films could be assembled into resistive-type pressure sensors by sandwiching the film between a copper foil and an indium tin oxide (ITO)-coated conductive flexible poly(ethyleneterephthalate) (PET) sheet. The resulting square pressure-sensitive pad was 1 cm 2 in size. Figure 2b depicts the piezoresistive response and the sensitivity of the device, which was monitored using methods depicted in Supplementary Fig. S8 . The pressure sensitivity S can be defined as the slope of the resistance versus pressure in Fig. 2b ( S = dR / dp ), where R denotes the resistance and P denotes the applied pressure. The resistance versus pressure curve revealed a similar power law dependence of sensitivity on pressure. In the <100 Pa pressure range, the device showed ultra-high sensitivity of ~7.7–41.9 kPa −1 . At pressures >1 kPa, the sensitivity dropped to <0.4 kPa −1 . The dependence of log R on log P and log S on log P was linear over a wide pressure range extending to 100 kPa ( Supplementary Fig. S9 ), in contrast, our capacitive pressure sensors based on organic thin film transistors showed an abrupt change of sensitivity at 2 (ref. 7 ) and 8 kPa (ref. 10 ). In real-world applications, a constant mathematical power law relationship between S and P is desirable because the progressive reduction of S allows for ultra-high sensitivity at very low loads and a large range of detectable pressures at higher loads (for which high sensitivity is not required). Our device exhibited an immediate response to both external loading and unloading, as shown in Fig. 2c , with response and relaxation times faster than ~50 ms, which was the resolution limit of our measurement system. Contact resistance mechanism of EMCP piezoresistance Further investigation revealed that these pressure sensors operate mainly through a contact resistance mechanism, i.e., the piezoresistance originates from physical contacts at discrete spots between the asperities of the EMCP film and the electrode surface [41] . To confirm the piezoresistance mechanism, we utilized a lateral device structure with ‘bottom contact’ geometry ( Supplementary Fig. S10a ), in which both of the electrodes were below the PPy film. The operation of the devices with and without contact resistance was compared. When the EMCP film was placed on the electrodes, a large change in resistance was observed with increasing pressure. However, after the contact resistance was eliminated by adhering the EMCP film to the electrodes through a wetting and heat treatment process, the resistance was effectively constant with applied pressure (see Supplementary Fig. S10b and Supplementary Note 1 for more information), indicating the piezoresistance can be attributed to the contact resistance between the interfaces of the EMCP film and the electrode. This observation is consistent with previous research, which showed that PPy displayed little bulk piezoresistance [42] , [43] . Moreover, the inverse linear relationship between log R and log P displayed by our device ( Fig. 2b ) was consistent with the contact resistance equation [41] , [44] . Where R c denotes the contact resistance, ρ is the electrical resistivity and η is an empirical coefficient of order unity, H is the hardness of the material and F is the load [41] . It is generally accepted that the contact area is determined by the physical contact of the asperities projecting from the surface [45] . The contact area between EMCP and the electrode is directly proportional to the load and independent of the apparent area, enabling the sensing of an applied pressure. The spherical asperities of our EMCP thin film closely resemble the geometric model employed in the theoretical simulation of contact resistance [41] , [46] , [47] , resulting in a perfect inverse linear relationship between log R and log P . Research has shown that the magnitude of the contact resistance is significantly influenced by the size and shape of the asperities [48] , [49] as well as asymmetry in the resistivities of the two materials [50] , [51] . Our results comparing various top electrodes in the sandwich structure revealed that the roughness of the electrode had a large effect on the shape of the resistance versus pressure curve and the magnitude of the contact resistance ( Supplementary Fig. S11 ), implying the pressure sensing of EMCP could be tuned by controlling the interface roughness. It is worth noting that the elasticity of the EMCP film played an important role in stabilizing the sensing performance of the sensor. Our control experiment demonstrated that a device made of solid PPy particles exhibits poor and unstable piezoresistance ( Supplementary Fig. S12 ). Furthermore, research by McBride and coworkers demonstrated that the contact resistance of smooth, unstructured films of polyaniline resulted in unstable, immeasurable values of the contact resistance at low pressures [52] . Previously, pressure sensors based on contact resistance suffered from an inadequate working range [19] , large threshold values for accurate measurements [24] , [25] , [35] and unstable contact between electrode interfaces [53] . Our pressure sensor displays excellent performance with moderate hysteresis ( Fig. 2d ), reproducible cycling to 8,000 cycles between 0 Pa and 5 kPa ( Fig. 2e ) and consistent results at a range of loading speeds ( Supplementary Fig. S13 ). Moreover, the performance of our devices was highly reproducible, with six different devices exhibiting similar piezoresistive behaviour ( Supplementary Fig. S14a ). The elasticity of our EMCP film may play an important role in evenly distributing the pressure and accommodating the deformation; thus, stabilizing the contact between electrode interfaces. Stability with temperature and time Owing to the mechanism of contact resistance, the pressure response of our devices displayed only a slight dependence on ambient temperature. Because the piezoresistance is determined by the physical contact between the electrode interfaces, the devices’ sensing characteristics are not affected by the thermal expansion of the bulk. The temperature-dependent piezoresistance of the device is depicted in Fig. 2f . The device was tested with loadings of 8.16 and 22.45 Pa at a temperature range of –10 °C to 100 °C and exhibited only a slight signal drift as a function of temperature, showing the potential of our device to work in harsh-temperature ambient environments. The temperature stability of PPy was promoted by the use of non-volatile dopants, which are difficult to remove [54] , [55] and provide stable conductivities at temperatures of over 100 °C [54] . Our use of phytic acid (a high-molecular weight non-violatile dopant, MW=660.4 g mol −1 ) likely enabled the excellent temperature stability of our device. Moreover, a crosslinking effect may further promote temperature stability; each phytic acid molecule interacts with more than one PPy chain. The excellent temperature stability we observed is in contrast to devices based on bulk piezoresistance, which often exhibit changes in conductivity of up to an order of magnitude within the same temperature range [56] , [57] . In addition to desirable temperature response, our highly stable phytic acid dopants also contribute to good stability over time. Devices using EMCP films measured after 10 months of storage showed similar characteristics ( Supplementary Figs S14 and S15 ), with an average increase in resistance of 77%. In contrast, a dramatic increase in the resistance of PPy with time has been observed in other reports and was accelerated by exposure to air [58] , [59] , which resulted in an increase in resistivity by 3–5 times over 1 month in ambient condition. The device stability should be further improved by using better encapsulating methods. Enhanced piezoresistance sensing by patterning EMCP The sensitivity of our pressure sensor can be further improved by adapting the microstructuring strategy we used previously for capacitive pressure sensors by patterning the surface of the EMCP thin film [7] . The microstructured surface was fabricated by moudling a surface topology (lines with a triangular cross-section profile with 0.5 mm height and 1 mm width) onto PPy films before gelling, as shown in Fig. 3a . The PPy hydrogel replicated the microstructures regularly and uniformly across the full size of the wafer mold. 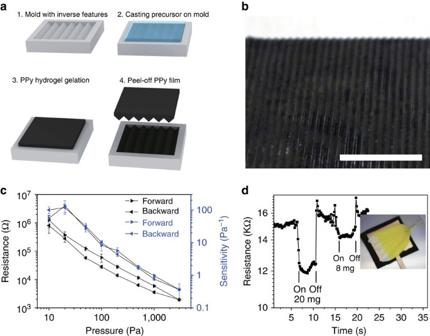Figure 3: Fabrication and resistive pressure response of micropatterned EMCP films. (a) Schematic process for the fabrication of micropatterned EMCP films. The precursor solution of the PPy gel was drop cast on the mold (step 1) containing arrays of the features to be replicated (step 2). The solution gelled quickly (step 3). After the purification process, the PPy hydrogel film was frozen and peeled-off the mold (step 4). (b) Digital photo image of the micropatterned PPy film. (c) Resistance response and pressure sensitivity of the EMCP pressure sensor, scale bar: 1 cm. The error bars represent one standard deviation. (d) Transient response to the application and removal of a 20 mg weight and a flower petal (8 mg) on the micropatterned EMCP device, the latter corresponding to a pressure of only 0.8 Pa. Figure 3b shows the piezoresistive response to pressure of the patterned EMCP device. The microstructured EMCP film displayed a markedly increased sensitivity ( Supplementary Fig. S16 ) compared with the unstructured film and retained a linear relationship between log R and log P . To our knowledge, the sensitivity (~56.0–133.1 kPa −1 ) of our device in the low-pressure regime (<30 Pa) is the highest reported, and the device is far more sensitive than the subtle pressure sensing properties of natural human skin. The patterned PPy film reliably detected the placement and removal of a tiny weight such as a flower petal (weight: 8 mg), as shown in Fig. 3d , which corresponds to an extremely low pressure of 0.8 Pa, making our device more sensitive than our microstructured PDMS capacitive pressure sensor (3 Pa) [7] and the interlocking nanowire-type pressure sensor (5 Pa) [19] . High sensitivity in a device assembly can be retained using two general methods. The first is to use elastic spacers to control the contact between the two electrodes in the encapsulated devices ( Supplementary Fig. S17b and c ). The spacers can be insulating polymer bars, dots or a mesh [35] . The second method is to engineer the electrode surface with high roughness to retain high sensitivity over a larger pressure range so that a small preload will not be detrimental to the device sensing properties [60] . The alternative is microstructuring of the PPy layer as what we have shown in this paper. Figure 3: Fabrication and resistive pressure response of micropatterned EMCP films. ( a ) Schematic process for the fabrication of micropatterned EMCP films. The precursor solution of the PPy gel was drop cast on the mold (step 1) containing arrays of the features to be replicated (step 2). The solution gelled quickly (step 3). After the purification process, the PPy hydrogel film was frozen and peeled-off the mold (step 4). ( b ) Digital photo image of the micropatterned PPy film. ( c ) Resistance response and pressure sensitivity of the EMCP pressure sensor, scale bar: 1 cm. The error bars represent one standard deviation. ( d ) Transient response to the application and removal of a 20 mg weight and a flower petal (8 mg) on the micropatterned EMCP device, the latter corresponding to a pressure of only 0.8 Pa. Full size image Prototype circuit of pressure sensor arrays For human–computer interfaces applications, it is desirable to scale up the sensor to an array configuration of several pixels to collect spatially resolved pressure information. Employing the EMCP films, we fabricated a proof-of-concept resistive pressure sensor matrix of 64 pixels on a chess board. Each of the pixels measured ~36 mm 2 . The sensor array monitored the weight distribution on each pixel by detecting the pixel resistance. Supplementary Movie 1 shows the rapid response in resistance when loading and unloading the chess pieces on one of the pixels. A specific weight can be added specifically to the black chess pieces to make them have different weight with white analogues to enable the identification of the colour of pieces on the chess board. 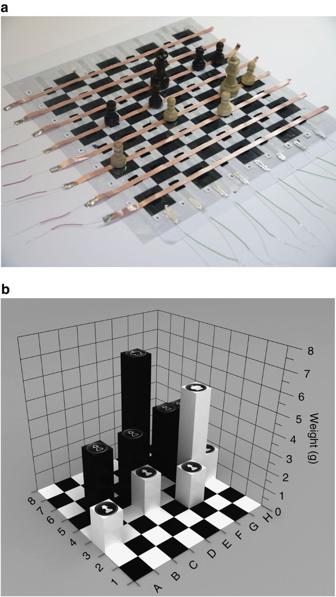Figure 4: A prototype pressure sensor on a chess board. (a) A real-world chess board with pieces distributed on the pressure sensor array. (b) Reconstructed map with columns labelled with the piece identities and with their heights corresponding to the calibrated weights (the sensor pixels were calibrated against two known weights). Figure 4a depicts a chess board, in which the position and the type of the pieces on the chess board were identified by measuring their weights as shown in Fig. 4b on a reconstructed map in which the height of each pixel bar corresponds to the calibrated weight of the chess piece (listed in Supplementary Table S1 , calibrated against two known weights on each pixel). This matrix of pressure sensors demonstrate the potential for applying our sensor networks in human–electronics interfaces and electronic skin devices. Figure 4: A prototype pressure sensor on a chess board. ( a ) A real-world chess board with pieces distributed on the pressure sensor array. ( b ) Reconstructed map with columns labelled with the piece identities and with their heights corresponding to the calibrated weights (the sensor pixels were calibrated against two known weights). Full size image We present a new material design concept to impart elasticity to a rigid conducting polymer by forming hollow-sphere microstructures. Even conjugated polymers can be made flexible by introduce alkyl side groups; however, conducting polymers are usually non-compressible. Herein, we were able to prepare an EMCP with hollow-sphere structures through a novel multiphase synthesis strategy. The facile solution gelation synthesis allowed us to fabricate and pattern large area EMCP thin films through casting process easily. Such gelation mechanisms are compatible with other large scale patterning technologies such as ink-jet printing or spray coating [61] . The interconnected hollow-sphere structure enabled the conducting PPy elastically deform and recover upon the application and release of external pressure. The EMCP enabled us to build a new type of resistive pressure sensor based on a contact-resistance mechanism. This solved the common problems usually associated with resistive pressure sensors working on bulk-piezoresistance effect and achieved high sensitivity, low threshold, low hysteresis, excellent cyclability and temperature-stable sensing. The pressure sensor exhibited unprecedented performance with ultra-high sensitivity. By patterning the surface of the EMCP thin film, the sensitivity of our pressure sensor can be ultimately improved to ~56.0–133.1 kPa −1 in the low-pressure regime (<30 Pa), the highest among any reported flexible pressure sensors (for comparison, 0.55 kPa −1 in 0.2 kPa range in Mannsfeld et al . [7] , and 8.2 kPa −1 in Schwartz et al . [10] ). Moreover, our pressure sensor was able to detect the placement or removal of a tiny weight such as a flower petal corresponding to an extremely low pressure of 0.8 Pa. Notably, the elasticity induced by hollow-sphere microstructure of the PPy, the key innovation of our material design, played an important role to impart the device with stable electrode contact, reproducible cycling and temperature stable sensing performance sensing features. In summary, the rigid conductive polymer PPy is fashioned into films composed of hollow-sphere microstructures, endowing the PPy with structure-derived elasticity and enabling rational designs for ultra-sensitive, rapid-responding and reliable pressure sensors. By harnessing the structure-derived elasticity and ultra-low effective elastic modulus of the EMCP material, our contact-resistance-type pressure sensor exhibits unprecedented pressure sensitivities. These EMCP-based contact-resistance-type pressure sensors, with the advantages of ultra-high sensitivity, a wide dynamic range, rapid response times and temperature-stable operation, will meet the application needs of a vast variety of fields, such as human–computer user interfaces, robotics, and industrial monitoring. Moreover, we foresee that EMCP materials will be highly useful in the design of next-generation electronic systems due to their advantageous traits, including a 3D hierarchical morphology, high conductivity, and good elasticity. Materials synthesis A 0.274 g (1.2 mmol) mass of ammonium per sulfate (Aldrich) was dissolved in 0.5 ml deionized water (DI) water (solution A). Solution B was prepared by mixing 84 μl pyrrole (99%, Aldrich) in 0.5 ml isopropanol, followed by 0.184 ml phytic acid (50%, wt % in water, Aldrich). The reaction vial and A/B solutions were rapidly cooled to roughly 4 °C using dry ice. The A and B solutions were then quickly mixed, cast into a Petri dish and allowed to react for 2 h. To remove excess ions, acid and by-products, the PPy gel thin film was further purified by sequential immersion in excess ethanol (12 h) and DI water (24 h). The PPy film was dried at 60 °C under vacuum and was rehydrated to form a hydrogel by adding DI water ( Supplementary Fig. S17 ). The dehydrated PPy film used for the device was prepared by drying in the ambient environment for 3 days. The patterned PPy film was prepared by casting the mixed precursor solution onto a PDMS mold with a 1-mm period and 0.5-mm height embossment. The patterned PPy hydrogel was peeled-off after freezing. Characterization The morphologies of the products were examined using field emission scanning electron microscopy (SEM, LEO 1530) and transmission electron microscopy (TEM, FEI, TECHNAI 20). Fourier transform infrared spectra were recorded on a NEXUS 870 spectrophotometer. Static contact angles were measured with an Edmund Scientific goniometer and milli-Q water was used as the probe fluid. The conductivity of the pressed sample pellets was measured using a standard four-point probe method at room temperature. The resistance was obtained using an Agilent E4980A Precision LCR metre. Pressure sensor cycling measurements were performed on a mechanized z axis stage (Newmark Systems, 0.1 mm resolution), and a force gauge (Mark 10) was used to apply loads to the sensor pads on a custom-built probe station. The mechanical properties of the material were characterized by applying a compressive load to an ~181 μm thick PPy film sandwiched between glass substrates with a high-resolution micromechanical testing system (Delaminator Test System, DTS). Pressure-sensing device fabrication The EMCP films were assembled into a resistive-type pressure sensor by sandwiching them between a copper foil and an ITO-coated conductive flexible PET sheet. The size of the square pressure-sensitive pad was 1 cm 2 . The devices used for cycling and temperature-dependent testing were encapsulated in a PET enclosure. ITO was used for both of the electrodes in the device used for the temperature-dependence experiments to avoid the large thermal expansion effect of copper electrodes. Measurement techniques for resistance versus pressure data The resistance versus pressure data was collected using two different measurement methods. Supplementary Figure S8a shows a method in which an EMCP was adhered to a bottom gold electrode. Subsequently, a copper electrode measuring 1 cm × 1 cm was placed on the stack and a glass slide measuring 1 cm × 1 cm was placed on the copper electrode to ensure even distribution of the force applied by the force gauge as the device stack was raised by a motorized stage. The resistance was measured between the top and bottom electrodes using an LCR metre. This measurement method was used to collect the data in Fig. 2d–f . Owing to the static force applied by the weight of the glass slide, the pressure response in the low-pressure regime (<100 Pa) is negligible. As the pressure applied by the force gauge was removed, the force acting on the interface between the copper and EMCP converged to that of the weight of the glass slide. As depicted in Supplementary Fig. S8b , the second measurement method involved securing a top copper or gold electrode to the force gauge. An EMCP adhered to a bottom gold electrode was raised by a motorized stage and pressed against the top electrode. This method was used to collect the data depicted in Figs 2b and 3c , Supplementary Figs S9, S11d, S12–S16 . Because of the lack of static pressure between the EMCP and the top electrode, this method allowed the measurement of contact resistance at small pressures. As observed by comparing Fig. 2b,d , in the region greater than 100 Pa, the two different measurement methods provide similar characteristics in terms of the magnitude of the changes in resistance and the exponent in the power law relationship. How to cite this article: Pan, L. et al . An ultra-sensitive resistive pressure sensor based on hollow-sphere microstructure induced elasticity in conducting polymer film. Nat. Commun. 5:3002 doi: 10.1038/ncomms4002 (2014).